The effectiveness of coral reefs for coastal hazard risk reduction and adaptation The world’s coastal zones are experiencing rapid development and an increase in storms and flooding. These hazards put coastal communities at heightened risk, which may increase with habitat loss. Here we analyse globally the role and cost effectiveness of coral reefs in risk reduction. Meta-analyses reveal that coral reefs provide substantial protection against natural hazards by reducing wave energy by an average of 97%. Reef crests alone dissipate most of this energy (86%). There are 100 million or more people who may receive risk reduction benefits from reefs or bear hazard mitigation and adaptation costs if reefs are degraded. We show that coral reefs can provide comparable wave attenuation benefits to artificial defences such as breakwaters, and reef defences can be enhanced cost effectively. Reefs face growing threats yet there is opportunity to guide adaptation and hazard mitigation investments towards reef restoration to strengthen this first line of coastal defence. Nearly 40% of the world’s population lives within 100 km of the coast and that percentage is increasing [1] . The growing natural hazards from coastal storms, flooding and rising sea level [2] create social, economic and ecological risks of global significance. The United Nations global report on disaster risk reduction identified that the risks of economic loss associated with floods and tropical cyclones are increasing across the world [3] . The proportion of the world’s Gross Domestic Product annually exposed to tropical cyclones increased from 3.6% in the 1970s to 4.3% in the first decade of the 2000s (ref. 3 ). Moreover, the impacts associated with inundation and flooding from sea-level rise and storms are expected to increase substantially. As a consequence, huge investments are being made in coastal hazard mitigation and increasingly in climate adaptation, and these investments are often for artificial defence structures such as seawalls and breakwaters. These costs will increase. For example, the cost of dikes alone is predicted to increase to US$ 12–71 billion per year by 2100 (ref. 4 ). In recent climate negotiations, developed nations pledged US$ 100 billion per year by 2020 to support mitigation and adaptation in developing countries many of which are tropical and coastal. Adaptation funds are already starting to flow from these commitments at US$ 1–4 billion per year [5] . Governments and businesses are increasingly interested in identifying where nature-based solutions can be used cost effectively as part of the strategy for coastal defence and as an alternative to investing solely in artificial defences [6] , [7] , [8] , [9] . There is a growing body of evidence that suggests that nature-based solutions can be effective for risk reduction [10] , [11] , [12] , [13] . This evidence is clearest for mangroves and marshes [10] , [11] , [12] , [13] , [14] , [15] , [16] . The evidence is less well developed for coral reefs, and there is not a synthesis of the role of reefs in risk reduction. A clear assessment of the role and effectiveness of coral reefs for hazard mitigation should inform investments in coastal defence and could encourage investments to enhance reef resilience. Understanding the role of coral reefs in coastal protection is critical as some analyses have suggested that reef structures and associated ecosystem services might collapse unless both local and global actions are taken to reverse their decline [17] . In the past, when reefs have been damaged following extensive coral mining or land reclamation then investments increased in artificial defences [18] , [19] , [20] . Here we provide the first global synthesis and meta-analysis of the contributions of coral reefs to risk reduction and adaptation. Our aims are to quantitatively assess the published evidence for the effects of reefs on wave attenuation and to examine which parts of the reef have been shown to have the greatest effects on wave attenuation; to determine where and how many at-risk people might receive risk reduction benefits from reefs; and to provide a physical and economic comparison of the risk reduction value of reefs relative to built infrastructure. Wave attenuation Our systematic literature search identified 255 studies on coral reefs and wave attenuation. We could extract data for meta-analyses from 27 independent publications that covered reefs across the Atlantic, Pacific and Indian Oceans to quantitatively estimate the effectiveness of coral reefs in wave attenuation. We examined available studies on wave attenuation across three reef environments: the reef crest, reef flat and the whole reef ( Fig. 1 ). The reef flat is the shallow part of the reef that extends outward from the shore. It is often characterized by reduced water circulation, the accumulation of sediments and periods of tidal emersion. The reef crest is the seaward edge and often the shallowest part of the reef, and where wave breaking first occurs. The transition between reef flat and reef crest can often be gradual. 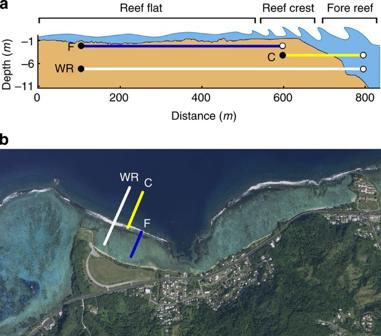Figure 1: Example of coral reef environments and sample transects. Transects along which wave attenuation was estimated for the three environments are indicated: reef flat (F), reef crest (C) and whole reef (WR). Measurements of wave parameters were compared between an offshore control (open circle) and a landward treatment (solid circle) in each transect. (a) Cross-section of the Camel Rock, Guam, fringing reef, from US Army Corps of Engineers SHOALS lidar data. (b) Aerial view of Asan Bay, Guam (data available from the US Geological Survey). We report the effects of reef crest, reef flat and whole reef separately, because only a few studies examined wave attenuation across all three environments, and we had to use data from sometimes different reefs for analyses by environment ( Supplementary Table 1 and Supplementary Methods ). Figure 1: Example of coral reef environments and sample transects. Transects along which wave attenuation was estimated for the three environments are indicated: reef flat (F), reef crest (C) and whole reef (WR). Measurements of wave parameters were compared between an offshore control (open circle) and a landward treatment (solid circle) in each transect. ( a ) Cross-section of the Camel Rock, Guam, fringing reef, from US Army Corps of Engineers SHOALS lidar data. ( b ) Aerial view of Asan Bay, Guam (data available from the US Geological Survey). Full size image Reefs significantly reduced wave energy across all three environments ( Fig. 2a and Supplementary Fig. 1a ). Reef crests dissipated on average 86% ( n =10; 95% confidence interval: 74–92%) of the incident wave energy ( Fig. 2a ). Reef flats dissipated 65% of the remaining wave energy ( n =23; 58–71%). The whole reef accounted for a total wave energy reduction of 97% ( n =13; 94–98%; Fig. 2a ). 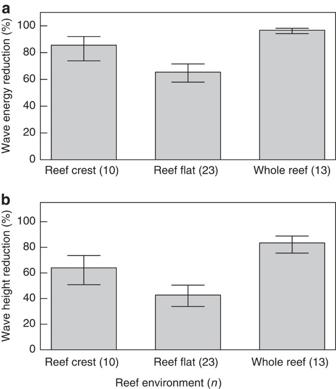Figure 2: Coral reef and wave attenuation meta-analysis results. Values are the average percentage of (a) wave energy reduction, and (b) wave height reduction in the three reef environments. Error bars represent 95% confidence interval. When the confidence intervals do not overlap, the averages are considered significantly different from zero (P<0.05). ‘n’reflects the number of independent experiments. Figure 2: Coral reef and wave attenuation meta-analysis results. Values are the average percentage of ( a ) wave energy reduction, and ( b ) wave height reduction in the three reef environments. Error bars represent 95% confidence interval. When the confidence intervals do not overlap, the averages are considered significantly different from zero ( P <0.05). ‘ n’ reflects the number of independent experiments. Full size image Reefs significantly reduced wave height across all three environments ( Fig. 2b and Supplementary Fig. 1b ). The reef crest reduced wave height by 64% ( n =10; 51–74%). The reef flat reduced wave height by 43% ( n =23; 34–51%; Fig. 2b ). The whole reef reduced wave height by 84% ( n =13; 76–89%; Fig. 2b ). We could extract data on wave type (that is, swell and wind waves) from only a subset of studies to examine if and how reefs reduced energy by wave type. Wave energy in both swell and wind wave types was reduced across all three environments (the whole reef, reef crest and reef flat) although not always significantly even when combined across experiments. Reef crests significantly dissipated 70% ( n =4; 43–84%) of the incident swell wave energy, and the whole reef significantly reduced both wind and swell wave energy ( Supplementary Fig. 2 ). Reef flats reduced both wind and swell wave energy, but our analysis of existing studies showed a significant effect only for swell waves ( Supplementary Fig. 2 ). The change in wave energy across the reef flat was much lower than across the reef crest or whole reef, which makes detection of individual wind wave effects more difficult. Using data on incident wave energy from reviewed studies, we also examined the relationship between maximum incident wave energy and wave energy reduction by reefs reported for each individual experiment ( Supplementary Table 2 ). The studies included in these analyses reported data recorded during different meteorological condition (calm to stormy), different seasons and for periods up to 4 consecutive months. Both reef crests and reef flats dissipated disproportionately more wave energy as incident wave energy increased ( Fig. 3 ). Nonlinear regressions indicated that for reef crests and reef flats, wave energy reduction reached asymptotes of 91% and 67%, respectively ( Fig. 3 ). The effects of the whole reef in dissipating wave energy were linear from small through hurricane-level waves, that is, the reefs reduced a consistent 97% percent of the incident wave energy ( Fig. 4 and Supplementary Fig. 3 ). 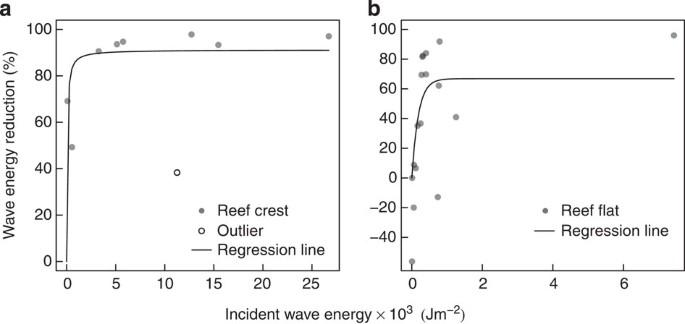Figure 3: Wave energy reduction as a function of maximum incident wave energy. The relationship was investigated across (a) reef crests (n= 9) and (b) reef flats (n=17). Only experiments for which data were available in J m−2were used. The asymptotic equations for the relationship between wave energy reduction (y) and maximum incident wave energy (x) at the reef crest and reef flat are (y=91.2/(1+52.4/x)) and (y=66.8 × [1−e(−x/185)]), respectively. The plottedxvalues are (J m−2× 103) for visual representation purposes, whereas in the equations they are simply in J m−2. Ina, the regression did not include the outlier (open circle) as reef crest was comparatively very deep (5 m, see Methods). Inb, exclusion of the point at maximum wave energy does not substantially change the regression line (for example, asymptote changes from 66.8 to 61.6). Figure 3: Wave energy reduction as a function of maximum incident wave energy. The relationship was investigated across ( a ) reef crests ( n = 9) and ( b ) reef flats ( n =17). Only experiments for which data were available in J m −2 were used. The asymptotic equations for the relationship between wave energy reduction ( y ) and maximum incident wave energy ( x ) at the reef crest and reef flat are ( y =91.2/(1+52.4/ x )) and ( y =66.8 × [1− e (− x /185) ]), respectively. The plotted x values are (J m −2 × 10 3 ) for visual representation purposes, whereas in the equations they are simply in J m −2 . In a , the regression did not include the outlier (open circle) as reef crest was comparatively very deep (5 m, see Methods). In b , exclusion of the point at maximum wave energy does not substantially change the regression line (for example, asymptote changes from 66.8 to 61.6). 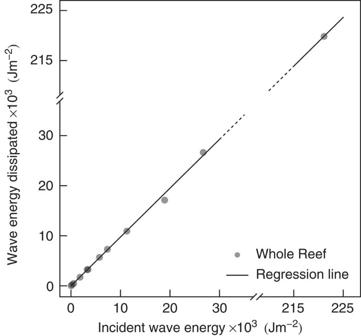Figure 4: Wave energy dissipated across the whole reefs as a function of maximum incident wave energy. Only experiments for which data were available in J m−2were used (n=12). Trend line for the linear regression is (y=0.97x;R2=0.9). Both thexaxis and the trend line have been broken to help the display the relationship across the full range of incident wave energy. Full size image Figure 4: Wave energy dissipated across the whole reefs as a function of maximum incident wave energy. Only experiments for which data were available in J m −2 were used ( n =12). Trend line for the linear regression is ( y =0.97 x ; R 2 =0.9). Both the x axis and the trend line have been broken to help the display the relationship across the full range of incident wave energy. Full size image After passing over the crest, waves were attenuated significantly across wider reef flats. However, most of the wave attenuation happened in the first part of the reef flat; 50% of the reduction in both wave energy and height occurred within <150 m from the reef crest in the experiments that we analysed ( Fig. 5 ). 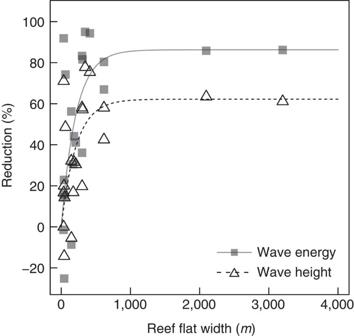Figure 5: The effects of reef flat width on wave attenuation. Percent reduction of both wave energy (n=21) and wave height (n=21) is reported as a function of coral reef flat width. Only experiments for which reef flat width was available were used. Each point is the percent wave attenuation for each experiment with trend lines (wave energy reduction:y=86.2 × [1−e(−x/210.2)]; and wave height reduction:y=62.2 × [1−e(−x/213.3)]). Figure 5: The effects of reef flat width on wave attenuation. Percent reduction of both wave energy ( n =21) and wave height ( n =21) is reported as a function of coral reef flat width. Only experiments for which reef flat width was available were used. Each point is the percent wave attenuation for each experiment with trend lines (wave energy reduction: y =86.2 × [1− e (− x /210.2) ]; and wave height reduction: y =62.2 × [1− e (− x /213.3) ]). Full size image Comparing coral reefs to artificial coastal defences The transmission coefficient, K t (that is, the ratio of the transmitted to the incident significant wave height H t / H i ), of low-crested detached breakwaters typically ranged from 0.3 to 0.7, which represents a wave height reduction of 30–70% (refs 21 , 22 , 23 , 24 , 25 ). This range is comparable to the one estimated from our meta-analysis for coral reefs (51–74%); the average wave height reduction for reefs (64%; Fig. 2b ) is in the upper range of values reported for artificial structures. The costs of building tropical breakwaters ranged between US$ 456 and 188,817 m −1 ( Table 1 ) with a median project cost of US$ 19,791 m −1 ( n= 16). The construction costs of structural coral reef restoration projects ranged between US$ 20 and 155,000 m −1 with a median project cost of US$ 1,290 m −1 ( n =13) ( Table 2 ). On average, the costs of the restoration projects were significantly cheaper than costs of building tropical breakwaters ( t -test: t (27) =3.762, P <0.001). Table 1 Costs of construction or significant maintenance intervention for tropical breakwaters. Full size table Table 2 Costs of coral reef restoration projects. Full size table Reefs and coastal populations We estimate that there are up to 197 million people that live both below 10 m elevation and within 50 km of a reef who may receive risk reduction benefits from reefs ( Fig. 6 and Table 3 ). If we consider only areas within 10 km of a reef (that is, an 80% reduction in distance) and below 10 m elevation, there are still some 100 million people who may receive risk reduction benefits from reefs ( Table 3 ). 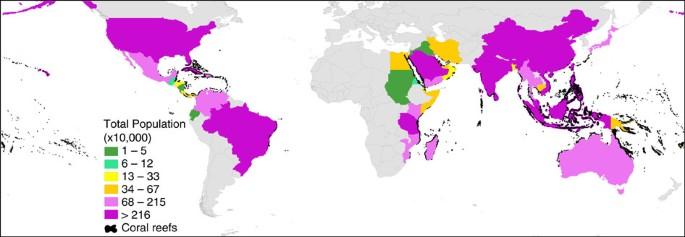Figure 6: The number of people who may receive risk reduction benefits from reefs by country. The countries are grouped by the number of people living below 10 m elevation and within 50 km of a coral reef as indicated in the legend. Countries in grey either have no data or no people meeting these conditions. Global and country maps are accessible fromwww.maps.coastalresilience.org. Figure 6: The number of people who may receive risk reduction benefits from reefs by country. The countries are grouped by the number of people living below 10 m elevation and within 50 km of a coral reef as indicated in the legend. Countries in grey either have no data or no people meeting these conditions. Global and country maps are accessible from www.maps.coastalresilience.org . Full size image Table 3 Number of people who may receive risk reduction benefits from coral reefs by country. Full size table The countries with the greatest number of at-risk people who may receive risk reduction benefits from reefs are Indonesia, India and the Philippines whether we consider distances of 10 or 50 km from reefs. These three countries alone include ~\n50% of the people globally that live in low exposed areas near reefs ( Table 3 ). The USA ranks within the top 10 of countries in number of people that may receive risk reduction benefits from reefs. We provide the first quantitative meta-analysis of the role of coral reefs in reducing wave energy across reefs in the Indian, Pacific and Atlantic Oceans. Combined results across studies show that coral reefs dissipate 97% of the wave energy that would otherwise impact shorelines. Most (86%) of the wave energy is dissipated by the reef crest; this relatively high and narrow geomorphological area is the most critical in providing wave attenuation benefits. The reef flat dissipates approximately half of the remaining wave energy, most of the wave energy on the reef flat is dissipated in the first part of the reef flat (that is, the 150 m closest to the reef crest). This means that even narrow reef flats effectively contribute to wave attenuation. These results are consistent with both models and observations of coastal barriers that identified cross-shore bathymetric profile, and in particular the height of the barrier (for example, reef crest), as the most important variable in coastal defence considerations [15] , [26] , [27] , [28] . The depth of reefs, particularly at the shallowest points, is critical in providing wave attenuation benefits. In order to better quantify these benefits in the future, much greater emphasis needs to be placed on measuring the depth profile including across tidal cycles and during events when water levels are raised (for example, storm surge). After bathymetry, another critical factor in wave attenuation is bottom friction, which is a function of bottom roughness [29] , [30] . Coral reef degradation has significant impacts on roughness. For example, the loss of branching Staghorn and Elkhorn corals ( Acropora spp.) Caribbean-wide affects both height and roughness particularly on reef crests [31] . Unfortunately, most studies included in our meta-analysis did not report information on species composition or rugosity. Better information on these factors would inform reef restoration and conservation efforts, because they would allow better identification of those species critical to delivering wave attenuation benefits. The whole reef dissipates energy with linear (that is, constant) effect from small through hurricane-level waves. The effect of the reef crest on wave reduction is nonlinear and intensifies as incident wave energy increases. These effects are critical for exposure reduction; reefs are relevant for risk reduction even during extreme events. For example, in 2005 during Hurricane Wilma incident wave heights reached 13 m and the Meso-American reef attenuated 99% of this height [32] . These data are also consistent with common observations (for example, surfing videos) that large waves (>7 m) break and dissipate most of their energy on reef crests [33] . We also showed that reefs are critical not just for low-frequency, high-energy events (for example, storms and cyclones), but by significantly reducing swell waves they reduce coastal erosion from the high-frequency (that is, daily) wave events. Storms are known to have negative short-term impacts on coral cover [34] , [35] , but reefs can be resilient and recover from these impacts [36] , [37] . Understanding when reefs (like any defence structure) fail during high-energy events and how long they take to recover is critical. These are parameters that can be reasonably measured and modelled if we take a cross-disciplinary approach to the engineering and ecology of reefs. Indeed, the role of reefs in coastal defence and how to restore these benefits needs to be addressed in greater detail, which will require greater collaboration among ecologists, engineers, geologists and oceanographers. Although coral reefs are one of the most well-studied marine ecosystems (for example, >18,000 papers on reef ecology and geology in the last 20 years), we found only 255 publications that even mentioned the role of reefs in wave attenuation, wave energy or wave breaking, and only 10% of these directly addressed the issue with data. By comparison, there were >5,000 papers that noted coral reef fish and fisheries. There are only a handful of studies of the implications of reef degradation for wave impacts on coastlines. In the Maldives, Red Sea, Cancun (Mexico) and Bali (Indonesia) there are inferred links between increases in coastal development, reef degradation and investments in artificial defences, but only a few direct studies on causality [18] , [19] , [20] , [38] , [39] . From a coastal engineering standpoint, any reef degradation (or sea-level rise) that increases water depth should result in more wave energy passing over the reef and through coastlines [39] . The loss of corals has led to real increases in wave energy reaching coastlines in the Maldives [39] . Based on our analyses and recent studies by the re-insurance industry [6] , we find that reef conservation and restoration can be cost effective for risk reduction and adaptation. In considerations of effectiveness, coral reefs can deliver wave attenuation benefits similar to or greater than artificial structures designed for coastal defence such as low-crested breakwaters. Trade-offs with other environmental considerations (for example, poor water quality in stagnant waters behind breakwaters) often require that artificial structures are designed to lower levels of effectiveness for coastal defence than is technically feasible [40] . We find that restoring reefs is significantly cheaper than building artificial breakwaters in tropical environments. Our findings are consistent with recent analyses from the re-insurance industry on the economics of climate adaptation across eight Caribbean nations [6] . They examined the costs and benefits of some 20 different approaches for coastal risk reduction and adaptation from reef restoration to new building codes. They found that reef restoration was always substantially more cost effective than breakwaters across all eight nations considering only coastal defence benefits. Moreover, reef restoration was one of the most cost effective of all approaches in seven of eight nations. A full benefit:cost analysis of coastal defence alternatives that includes coral reefs is desirable but not yet possible. For reef restoration and even for breakwaters, there needs to be better accounting for benefits such as fisheries and recreation. For reef restoration, there needs to be better accounting for maintenance costs and longer term measures of the success of restoration efforts. These measures should consider the effects of restored reef depth and roughness on wave attenuation, reef failure points during high-energy events, and the recovery time periods and costs after these events. Many gaps remain in designing reef restoration projects for hazard mitigation, as very few projects have explicitly tried to deliver benefits for both risk reduction and reef conservation. As living structures, reefs have the potential for self-repair and thus lower maintenance costs as compared with artificial structures, but reef restoration is still a comparatively new field. Most measures of reef restoration projects are limited to just the time period in which a project is constructed (that is, one funding cycle) particularly in developing countries where most reef restoration occurs. The addition of ecosystem benefits and considerations of maintenance costs in a full benefit:cost analysis would likely add to the relative cost effectiveness of reefs for coastal defence. Reefs face many growing pressures from development and climate change. Some scientists question their viability in future centuries [41] . This view has been criticized as too pessimistic [42] . In considering the future of reefs, it has been noted that reefs will not simply disappear, and the effects of climate change on reefs will be species and site-specific [42] . There will also be strong evolutionary pressure for adaptation of corals to climate change [43] . The resilience of coral reefs to climate change can be enhanced by removing other stressors [42] , [44] , [45] , [46] , [47] . Indeed, in many cases, local threats are more significant than climate change in terms of impacts to coral reefs, and these are more manageable threats (for example, blast fishing, overexploitation of grazers, pollution and sedimentation) [46] , [47] , [48] , [49] . It is also important to consider that the current loss of coral reefs is lower than the loss of other coastal habitats [50] , [51] , and reefs thus harbour significant opportunities for conservation and restoration. Coral reefs can be an effective first line of defence and these benefits are important for many nations. Nearly 200 million people may receive risk reduction benefits from reefs or bear costs if the reefs are lost or degraded. A greater appreciation of the risk reduction benefits from reefs should help motivate the local and global actions needed to maintain and restore these ecosystems and the services they provide. The link between actions (reef structures rebuilt) and measures (wave attenuation) can be direct and timely, which is often critical for adaptation and risk reduction investments. Our analysis of existing studies suggests that restoration for hazard mitigation and adaptation would be particularly cost effective when focused along the reef crest, where the greatest wave energy reduction can be achieved. A management focus on reefs with the goal of providing risk reduction and adaptation benefits, however, will require changes in conservation and disaster risk reduction approaches. Although conservation efforts are most often directed to more remote reefs, our results suggest that there should also be a focus on reefs closer to the people who will directly benefit from reef restoration and management. Disaster risk reduction managers will also have to focus more on prevention measures such as sustainable development and environmental conservation, both are widely recognized as important and cost effective but rarely acted upon [3] . Literature search To identify articles with sufficient quantitative data for assessing wave attenuation by coral reefs, we conducted a literature search using Web of Science (1900–2013, cutoff date 20 October 2013). We systematically searched the literature using a combination of the following keywords: ‘coral reef*’ with ‘wave attenuation*’, ‘wave energy’ and ‘wave breaking’. We based the keyword selection on the results of a wider preliminary literature search. We used meta-analysis to combine the results of independent experiments and to assess the magnitude and direction of the difference between pairs of treatment and control groups [52] . We identified studies examining wave attenuation at different sites aligned along a cross-reef transect from offshore (control) to onshore (treatment) ( Fig. 1 ). Detailed descriptions of the literature screening and characteristics of reef and waves in the considered studies are provided in the Supplementary Methods . Extensive data from the studies that we used in the analysis are provided in Supplementary Data 1 , 2 , 3 . Wave attenuation measures We assessed two response variables to US measure the wave attenuation service of coral reefs: wave energy reduction and wave height reduction. Wave energy reduction and wave height reduction are functionally related, and we analysed and provided data on both variables. Wave energy is the most critical factor governing coastal processes and is particularly influenced by water (reef) depth, wave breaking [53] , [54] , [55] , [56] and friction with the reef substrate [29] , [56] . However, wave height reduction is a more easily understood parameter and also used in many engineering applications; wave height reduction is particularly influenced when the water depth is equal to half the wavelength ( d = λ /2). The energy of a wave is a function of its height as follows: where E is the wave energy density (hereafter just energy), ρ is water density, g is gravitational acceleration and H is the significant wave height. For the sake of comparison, the wave height data were all converted to the common metric H 1/3 , that is, the significant wave height of the highest third of the waves ( Supplementary Methods ). Data extraction We estimated the influence of reefs on waves across three reef environments: crest, flat and whole reef ( Fig. 1 ). The effect of the reef crest on waves was estimated by extracting data from wave sensors along transects offshore (control) and inshore (treatment) of the reef crest (see Supplementary Methods for further explanation). The effect of the reef flat was assessed by comparing waves measured at points on the outer reef flat (control) to waves measured at points on the inner reef flat adjacent to the shoreline (treatment). The effect of the whole reef was estimated by comparing waves measured from the fore reef (control) to the inner reef flat adjacent to the shoreline (treatment). Whenever possible, we also examined effects by wave type, that is, swell (period=8–20 s) and wind (period=3–8 s) waves, as the energy impacting structures varies by wave type ( Supplementary Methods ). We were not able to analyse the relationship between wave attenuation and water depth, as explicit data on tidal elevations were not available from most studies. However, we note that all studies and thus our analyses included measurements covering multiple tidal cycles (and depths). We report reef and wave characteristics of considered studies in Supplementary Methods and Supplementary Fig. 4 . In studies that did provide some information on reef depth, the reef crest was always ≤2 m in depth, except in one case where the reef crest was comparatively very deep (~\n5 m). Meta-analysis We used a random effects model for the meta-analyses, as most sets of experiments were heterogeneous as determined by calculating, Q T (the total heterogeneity), and testing it against a χ 2 -distribution with n −1 degrees of freedom [52] . For each independent experiment, we calculated the effect size as the log-response ratio ( ln R ) and its corresponding weighting factor, calculated as the reciprocal of the variance under the random model ( Supplementary Methods ) [57] , [58] . The effect size was calculated by taking the natural logarithm of the ratio between the mean of treatment ( L , onshore) and the mean of control ( S , offshore): For each analysis (for example,, overall effects of reef crest on wave energy), the overall effect size ( ln R ) was calculated by summing the products ( ln R of each experiment × its weighting factor) and dividing by the sum of the weights [58] . The log-response ratio ( ln R ) is a commonly used measure of effect size. It expresses the size of the treatment effect as a proportion of the control [58] , which enables a clear assessment of the magnitude of the effects of reefs on wave attenuation. In addition, this measure of effect size ( ln R ) enables comparisons even when the data are in different units (for example, J m −2 and percentages). Finally, ln R can be easily converted to a percent reduction of wave energy or height using: We report the results as percent reduction for wave energy and wave height, and provide the overall log-response ratios in Supplementary Fig. 1 . For each response variable, we considered the overall effect size ( ln R ) to be statistically significant ( P <0.05) if its 95% confidence interval did not overlap zero. All the analyses were also run using the Hedge’s g -effect size, another common effect size in meta-analysis, to evaluate the robustness of the results ( Supplementary Methods , Supplementary Fig. 5 ). All analyses were done using R 2.11.1 (ref. 59 ). Incident wave energy, reef flat width and wave attenuation We examined whether the effects of coral reefs on wave attenuation were related to incident wave energy by analysing the relationship between the maximum wave energy at offshore control sites and the corresponding percentage wave energy reduction at inshore treatment sites for the three reef environments. Similarly, we examined whether wave attenuation was a function of the reef flat width (see also Supplementary Methods ). Comparing coral reefs to artificial coastal defences To compare the effectiveness and costs of artificial structures and coral reefs, we searched published literature (including grey literature) for wave attenuation and construction and restoration costs. To compare effectiveness in wave attenuation, we focused on submerged (low-crested) detached breakwaters because they are the most comparable artificial structures to coral reefs in terms of structure height and placement, that is, parallel and close to shore with a crest at or just below the water surface [21] . Low-crested structures are relatively rare in tropical environments, but they are common in Europe and growing in use elsewhere because of their lower visual and environmental (water quality) impacts as compared with traditional emergent breakwaters [40] . The wave attenuation efficiency of low-crested detached breakwaters is measured by the transmission coefficient K t , which is the ratio of the transmitted to the incident significant wave height ( H t / H i ). K t depends on design parameters such as crest freeboard, crest width and structure permeability [60] , as well as local wave height and period. We compared K t values between low-crested structures (from our literature search) and coral reefs (from the meta-analysis) to assess the effectiveness of these two classes of structure in attenuating waves. For cost comparisons, we compared the costs of building breakwaters with the costs of restoration of coral reef structures. We focused on breakwaters and reefs built in tropical environments, as construction costs are often different between temperate and tropical or island environments. For coral reefs, we only used projects that restored structures (for example, with reef rubble or concrete blocks) as opposed to projects that only restored coral species (for example, by transplanting corals). The breakwater estimates come largely from the US Army Corps of Engineers. To consistently compare costs between artificial defences and reef restoration, we converted figures to linear units (US$ m −1 ) to be indicative of the costs to enhance or protect lengths of shoreline ( Supplementary Methods ). Costs for building breakwaters were usually reported in linear units (US$ m −1 ), whereas coral reef restoration project costs were reported in terms of restored area (US$ m −2 ). To convert the restoration figures to a unit length l (m −1 ) of shoreline enhanced, we assumed that an enhancement for l =1 m of shoreline protection would require restoring a reef section that was 5 m wide by 2 m high by l =1 m (10 m 3 ) of length parallel to shore (Goreau and Hilbertz [61] use similar width and height figures for reef restoration for coastal protection). Many restoration projects used stone or cement structures (for example, blocks) that were ~\n1 m 3 and then reported costs (US$ m −2 ) of arraying structures in a single layer on a reef [62] . Thus, to obtain a reasonable proxy of costs per linear m of shoreline enhanced, we considered that restoring 10 m 3 would require 10 × the reported restoration cost per m 2 . We tested for differences between reef restoration and breakwater construction costs using a two sample t- test. Data were log transformed to meet normality and variance homogeneity requirements. Reefs and coastal populations We estimated the population that might receive risk reduction benefits from coral reefs by mapping and quantifying the number of people living in both low-lying areas below 10 m elevation and near reefs (for example, Supplementary Methods and Supplementary Fig. 6 ). We examined two different distances (10 and 50 km) from reefs in considering how many people might receive risk reduction benefits from reefs. In terms of risk reduction, we consider direct and indirect effects, but do so conservatively. The most direct exposure reduction benefits (for example, wave energy and flooding reduction) are often within just a few kilometres of reefs and the coast (for example, 10 km). However, the number of people who might benefit from the avoided replacement costs for coastal defence (that is, indirect exposure benefits) extends well beyond those living in frequently flooded areas; the populations bearing these coastal defence and replacement costs can include whole provinces or island nations. Further indirect risk reduction benefits include the effects from reduced population vulnerability because of the provision of livelihood opportunities (for example, coastal jobs at ports, hotels or markets) and food security. Typical examinations of global coastal populations consider areas 50 km from the coastline or all areas below 10 m elevation no matter how far inland [63] . All of our estimates of people who may receive risk reduction benefits from reefs use more conservative estimates of coastal populations, because our analyses look only at the intersection of people who are both in low exposed elevations and near reefs off the coast. How to cite this article: Ferrario, F. et al . The effectiveness of coral reefs for coastal hazard risk reduction and adaptation. Nat. Commun. 5:3794 doi: 10.1038/ncomms4794 (2014).